Immunologic and chemical targeting of the tight-junction protein Claudin-6 eliminates tumorigenic human pluripotent stem cells The tumorigenicity of human pluripotent stem cells is a major safety concern for their application in regenerative medicine. Here we identify the tight-junction protein Claudin-6 as a cell-surface-specific marker of human pluripotent stem cells that can be used to selectively remove Claudin-6-positive cells from mixed cultures. We show that Claudin-6 is absent in adult tissues but highly expressed in undifferentiated cells, where it is dispensable for human pluripotent stem cell survival and self-renewal. We use three different strategies to remove Claudin-6-positive cells from mixed cell populations: an antibody against Claudin-6; a cytotoxin-conjugated antibody that selectively targets undifferentiated cells; and Clostridium perfringens enterotoxin, a toxin that binds several Claudins, including Claudin-6, and efficiently kills undifferentiated cells, thus eliminating the tumorigenic potential of human pluripotent stem cell-containing cultures. This work provides a proof of concept for the use of Claudin-6 to eliminate residual undifferentiated human pluripotent stem cells from culture, highlighting a strategy that may increase the safety of human pluripotent stem cell-based cell therapies. Human pluripotent stem cells (hPSCs) are a promising source of cells for regenerative medicine because of their unique self-renewal and differentiation properties [1] , [2] . However, safety concerns arise from their ability to generate tumours [3] . Previous studies have shown that residual hPSCs in differentiated populations can result in teratoma formation [4] , [5] , and it is thus important to eliminate all residual pluripotent cells before the clinical application of their derivatives. Importantly, the risk of teratoma formation is a major concern that is relevant both for human embryonic stem cells (hESCs) and for human-induced pluripotent stem cells (hiPSCs) [3] , [6] , [7] , and several strategies have been suggested to cope with this risk [8] , [9] , [10] , [11] . Cell surface markers of hPSCs can be invaluable for the selective removal of undifferentiated hPSCs from differentiated cultures [10] , [12] , [13] . Sorting out hPSCs using antibodies against cell surface antigens was previously performed to separate undifferentiated cells from heterogeneous cell populations to prevent teratoma formation [12] , [13] . Unfortunately, a single marker-based cell sorting was so far insufficient to completely eliminate undifferentiated cells and prevent teratoma formation [13] . A well-characterized pluripotent-specific cell surface protein may thus allow the selective immunologic or chemical targeting of undifferentiated cells. We therefore aimed to identify novel cell surface proteins that are uniquely expressed in hESCs and hiPSCs. By comparing a large data set of expression microarrays from various undifferentiated and differentiated cell types, we reveal that the tight-junction protein Claudin-6 (CLDN-6) is highly specific to pluripotent cells. Using the pluripotent-specific expression of CLDN-6 in hPSCs, we explore various strategies for the elimination of these cells from culture. We find that CLDN-6 targeting can remove hPSCs from culture in a rapid, robust and efficient manner, thus preventing teratoma formation from undifferentiated cells. CLDN-6 is selectively expressed in hPSCs To identify proteins that are uniquely expressed on the surface of human pluripotent cells, we first compared global gene expression patterns between undifferentiated and differentiated cells. Gene expression microarrays were performed with undifferentiated hESCs, undifferentiated hiPSCs, 30-day-old teratomas and 21-day-old embryoid bodies (EBs) differentiated from these hiPSCs, and the fibroblasts used for the hiPSC derivation. Global gene expression patterns were compared with each other, and to a reference expression data set from 11 human adult tissues ( Supplementary Table S1 ). Using the cellular component gene ontology (GO annotation), we searched for cell surface proteins that are expressed at least 10-fold higher in undifferentiated cells in comparison with all differentiated cell types. Only two genes met these stringent criteria: TDGF-1 and CLDN-6 ( Fig. 1a ). While TDGF-1 is a well-known marker of hPSCs [14] , [15] , CLDN-6 is a novel marker for these cells. CLDN-6 is highly specific to hPSCs, as its average expression in undifferentiated cells is ~90-fold compared with its average expression in differentiated tissues ( Fig. 1a ). Of note, CLDN-6 is more specific to hPSCs than many previously described pluripotent-specific surface proteins ( Fig. 1a ). To examine more comprehensively the expression of CLDN-6 across all human cell types, we queried the Amazonia expression atlas [16] . We found that CLDN-6 is indeed highly expressed in various hESC and hiPSC lines, as well as in human embryonic carcinoma cell lines, but is absent in over 250 samples of somatic tissues ( Fig. 1b ). 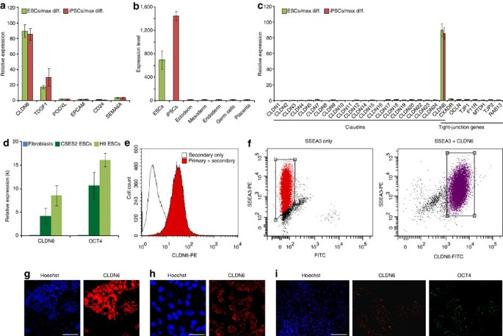Figure 1: Claudin-6 is uniquely expressed in human pluripotent stem cells. (a) Relative gene expression of the tight-junction protein CLDN-6 and several other pluripotent cell surface markers. Microarray expression level of each gene is compared between hESCs/hiPSCs and the adult tissue that shows the highest expression of that gene. (b) CLDN-6 expression in undifferentiated hPSCs and in various other human tissues (based on Amazonia expression atlas visualization for probeset 208474_at). Ectoderm includes brain, spinal cord, pituitary, adrenal, skin and mammary gland cells; mesoderm includes kidney, heart, adipose, prostate, testis, ovary, spleen, muscle, uterus, fibroblasts and blood cells; endoderm includes lung, stomach, intestine, colon, liver, pancreas, trachea and thyroid cells. (c) Relative gene expression of the Claudin family members and of several other tight-junction genes. (d) RT–PCR expression of CLDN-6 and OCT-4 in two hESC lines and in BJ fibroblasts. Fora–d, error bars indicate s.d. of the mean.n=3. (e) FACS analysis of undifferentiated hESCs shows the ubiquitous CLDN-6 expression in these cells. (f) FACS analysis of undifferentiated hESCs shows coexpression of CLDN-6 with the pluripotency marker SSEA-3. (g) Fluorescence microscopy imaging of undifferentiated hiPSCs immunostained with an antibody against CLDN-6 shows that all of them express CLDN-6, whereas the mouse embryonic fibroblasts that surround the colonies do not. Scale bar, 100 μm. (h) Confocal microscopy imaging of undifferentiated hiPSCs immunostained with an antibody against CLDN-6 shows that this protein is expressed on the membrane surface. Scale bar, 25 μm. (i) Microscopy imaging of undifferentiated hESCs immunostained with antibodies against OCT-4 and CLDN-6 shows coexpression of these proteins. Scale bar, 200 μm; diff., differentiated. Figure 1: Claudin-6 is uniquely expressed in human pluripotent stem cells. ( a ) Relative gene expression of the tight-junction protein CLDN-6 and several other pluripotent cell surface markers. Microarray expression level of each gene is compared between hESCs/hiPSCs and the adult tissue that shows the highest expression of that gene. ( b ) CLDN-6 expression in undifferentiated hPSCs and in various other human tissues (based on Amazonia expression atlas visualization for probeset 208474_at). Ectoderm includes brain, spinal cord, pituitary, adrenal, skin and mammary gland cells; mesoderm includes kidney, heart, adipose, prostate, testis, ovary, spleen, muscle, uterus, fibroblasts and blood cells; endoderm includes lung, stomach, intestine, colon, liver, pancreas, trachea and thyroid cells. ( c ) Relative gene expression of the Claudin family members and of several other tight-junction genes. ( d ) RT–PCR expression of CLDN-6 and OCT-4 in two hESC lines and in BJ fibroblasts. For a – d , error bars indicate s.d. of the mean. n =3. ( e ) FACS analysis of undifferentiated hESCs shows the ubiquitous CLDN-6 expression in these cells. ( f ) FACS analysis of undifferentiated hESCs shows coexpression of CLDN-6 with the pluripotency marker SSEA-3. ( g ) Fluorescence microscopy imaging of undifferentiated hiPSCs immunostained with an antibody against CLDN-6 shows that all of them express CLDN-6, whereas the mouse embryonic fibroblasts that surround the colonies do not. Scale bar, 100 μm. ( h ) Confocal microscopy imaging of undifferentiated hiPSCs immunostained with an antibody against CLDN-6 shows that this protein is expressed on the membrane surface. Scale bar, 25 μm. ( i ) Microscopy imaging of undifferentiated hESCs immunostained with antibodies against OCT-4 and CLDN-6 shows coexpression of these proteins. Scale bar, 200 μm; diff., differentiated. Full size image The Claudin family consists of 24 proteins that are essential for the formation of tight junctions in epithelial and endothelial cells. Different members of the family confer distinct properties to tight junctions, contributing to the diversity of these cellular barriers [17] . We therefore compared the expression of the family members between differentiated and undifferentiated cells, and found that CLDN-6 is the only pluripotent-specific Claudin ( Fig. 1c and Supplementary Fig. S1a ). Comparison with other tight-junction genes (from other protein families) revealed that CLDN-6 is the only differentially expressed tight-junction gene in hPSCs ( Fig. 1c ). To experimentally validate the data from the gene expression analysis, we directly tested the messenger RNA (mRNA) and protein levels of CLDN-6 in several hESC and hiPSC lines: RT–PCR (PCR with reverse transcription) analysis confirmed that CLDN-6 mRNA levels are extremely high in hESCs relative to differentiated BJ fibroblasts, and are comparable to those of the hallmark pluripotency gene OCT-4 ( Fig. 1d ); fluorescence-activated cell sorting (FACS) analysis with an antibody against human CLDN-6 showed that virtually all the cells in undifferentiated cultures express the protein ( Fig. 1e ), and that cells that express the well-known pluripotent markers SSEA-3 and TRA-1-60 coexpress CLDN-6 ( Fig. 1f and Supplementary Fig. S1b ); immunofluorescence staining validated that CLDN-6 is selectively expressed in undifferentiated hESCs and hiPSCs ( Fig. 1g ), that it is expressed on the membrane surface of the cells ( Fig. 1h ), and that OCT-4-positive cells are always CLDN-6-positive as well ( Fig. 1i ). We therefore conclude that CLDN-6 is a novel cell surface marker of hPSCs. CLDN-6 is not essential for hPSC survival and self-renewal Although CLDN-6 is selectively expressed in hPSCs compared with normal adult tissues, it was previously implicated in breast and gastric carcinomas, where its aberrant regulation could lead to anchorage-independent growth, increased invasiveness and apoptotic resistance [18] , [19] . Recently, CLDN-6 was also found to be expressed in germ cell tumours, and suggested to be a marker of cancers with a primitive phenotype [20] . In mouse development, Cldn-6 was recently found to be expressed in pluripotent stem cells [21] , and was also found to be important for endodermal development and epithelialization [22] , [23] . In human development, mild expression of CLDN-6 was recently observed in developing human epithelial structures during early- to-mid-gestation [20] , whereas its expression and role in hPSCs have not been explored. To examine whether inhibition of CLDN-6 would be sufficient for the elimination of hPSCs from culture, we knocked down endogenous CLDN-6 in undifferentiated hESCs. Targeting CLDN-6 with specific short interfering RNA resulted in >80% and >90% downregulation at the mRNA and protein levels, respectively ( Supplementary Fig. S2a,b ). However, the knockdown of CLDN-6 did not affect the morphology of the cells, and did not result in their differentiation, as was confirmed by RT–PCR and FACS analyses with pluripotency markers ( Supplementary Fig. S2c,d ). Moreover, CLDN-6 knockdown did not induce apoptosis in the cells ( Supplementary Fig. S2e,f ), and did not alter their cell cycle profile ( Supplementary Fig. S2g ). These data indicate that CLDN-6 is dispensable for the survival and self-renewal of hPSCs, consistently with previous data from the mouse: Cldn-6 knockout mice appeared phenotypically normal [23] , and knockdown of Cldn-6 in mouse ESCs did not compromise their pluripotency [21] . CLDN-6 is rapidly downregulated during hPSC differentiation As shown above, we identified the tight-junction protein CLDN-6 as a highly specific cell surface marker of hPSCs. Of note, while CLDN-6 is not detectable in adult tissues, it is still present in developing endodermal epithelia [20] , in line with its role in mouse embryonic development of endodermal tissues [22] , [23] . To examine how rapidly CLDN-6 is downregulated on differentiation of hPSCs into various lineages, we examined its expression in spontaneous and directed differentiation protocols. This analysis shows that CLDN-6 is significantly downregulated during the first 2 weeks of directed differentiation into the neural or cardiac lineages, but is still highly expressed in hPSC-derived hepatic and pancreatic progenitor cells ( Fig. 2a–e ). 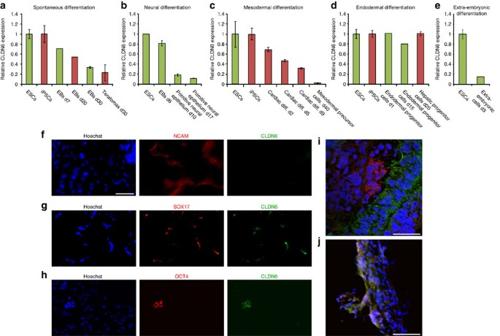Figure 2: Downregulation of CLDN-6 expression during hPSC differentiation. (a–e) Relative expression values of CLDN-6 throughout spontaneous and directed differentiation protocols of hESCs and hiPSCs. (a) Spontaneous differentiation into embryoid bodies or teratomas. Data are from the expression arrays used in the current study.n=3, 4, 1, 1, 2 and 3 for ESCs, iPSCs, EBs d7, EBs d20, EBs d30 and teratomas d30, respectively. (b) Directed differentiation into neural precursor cells. Data are derived from the NCBI Gene Expression Omnibus (GEO) database, accession number GSE9940.n=1, 2, 2 and 2 for ESCs, EBs d6, neural epithelium d10 and neural epithelium d17, respectively. (c) Directed differentiation into cardiomyocytes or mesodermal precursor cells. Data are derived from the GEO database, accession numbers GSE28191 and GSE7214 (ref.35).n=9, 2, 2, 2, 2 and 9 for ESCs, iPSCs, cardiac differentiation d2, cardiac differentiation d5, cardiac differentiation d9 and mesodermal precursors d40, respectively. (d) Directed differentiation into hepatic or pancreatic progenitor cells. Data of pancreatic differentiation are from ref.36; data of hepatic differentiation are derived from the GEO database, accession number GSE14897 (ref.37).n=3, 3, 1, 1 and 3 for ESCs, iPSCs, endodermal progenitors d1, endodermal progenitors d15 and hepatic progenitors d20, respectively. (e) Differentiation into extraembryonic (EPOR+) cells. Data are from ref.32.n=3 and 1 for ESCs and extraembryonic cells, respectively. In all cases (a–e), the expression levels are compared with those of the undifferentiated cells used for differentiation in the respective study. The bars are colour coded, so that green bars indicate differentiation from hESCs, whereas red bars indicate differentiation from hiPSCs. Error bars indicate s.d. of the mean. (f–h) Immunostaining of 14-day-old dissociated embryoid bodies with antibodies against CLDN-6 (in green) and NCAM (f), SOX-17 (g) or OCT-4 (h) (in red). Nuclei are stained with Hoechst 33342 (in blue). Scale bar, 100μm. (i–j) Immunostaining of teratoma sections with antibodies against CLDN-6 (in green) and NCAM (i) or SOX-17 (j) (in red). Nuclei are stained with Hoechst 33342 (in blue). Scale bars, 25 μm and 50 μm, respectively. diff., differentiated. Figure 2: Downregulation of CLDN-6 expression during hPSC differentiation. ( a – e ) Relative expression values of CLDN-6 throughout spontaneous and directed differentiation protocols of hESCs and hiPSCs. ( a ) Spontaneous differentiation into embryoid bodies or teratomas. Data are from the expression arrays used in the current study. n =3, 4, 1, 1, 2 and 3 for ESCs, iPSCs, EBs d7, EBs d20, EBs d30 and teratomas d30, respectively. ( b ) Directed differentiation into neural precursor cells. Data are derived from the NCBI Gene Expression Omnibus (GEO) database, accession number GSE9940. n =1, 2, 2 and 2 for ESCs, EBs d6, neural epithelium d10 and neural epithelium d17, respectively. ( c ) Directed differentiation into cardiomyocytes or mesodermal precursor cells. Data are derived from the GEO database, accession numbers GSE28191 and GSE7214 (ref. 35 ). n =9, 2, 2, 2, 2 and 9 for ESCs, iPSCs, cardiac differentiation d2, cardiac differentiation d5, cardiac differentiation d9 and mesodermal precursors d40, respectively. ( d ) Directed differentiation into hepatic or pancreatic progenitor cells. Data of pancreatic differentiation are from ref. 36 ; data of hepatic differentiation are derived from the GEO database, accession number GSE14897 (ref. 37 ). n =3, 3, 1, 1 and 3 for ESCs, iPSCs, endodermal progenitors d1, endodermal progenitors d15 and hepatic progenitors d20, respectively. ( e ) Differentiation into extraembryonic (EPOR+) cells. Data are from ref. 32 . n =3 and 1 for ESCs and extraembryonic cells, respectively. In all cases ( a – e ), the expression levels are compared with those of the undifferentiated cells used for differentiation in the respective study. The bars are colour coded, so that green bars indicate differentiation from hESCs, whereas red bars indicate differentiation from hiPSCs. Error bars indicate s.d. of the mean. ( f – h ) Immunostaining of 14-day-old dissociated embryoid bodies with antibodies against CLDN-6 (in green) and NCAM ( f ), SOX-17 ( g ) or OCT-4 ( h ) (in red). Nuclei are stained with Hoechst 33342 (in blue). Scale bar, 100μm. ( i – j ) Immunostaining of teratoma sections with antibodies against CLDN-6 (in green) and NCAM ( i ) or SOX-17 ( j ) (in red). Nuclei are stained with Hoechst 33342 (in blue). Scale bars, 25 μm and 50 μm, respectively. diff., differentiated. Full size image To further explore CLDN-6 downregulation during hPSC differentiation, we generated EBs from hESCs, dissociated and immunostained them after 2 weeks with antibodies against CLDN-6, together with antibodies against the hallmark pluripotency marker OCT-4, the neural progenitor marker NCAM or the endodermal progenitor marker SOX-17. In line with the microarray data, NCAM-positive cells did not express CLDN-6 ( Fig. 2f ), whereas many SOX-17-positive cells did express it ( Fig. 2g ). Rare residual undifferentiated cells coexpressed OCT-4 and CLDN-6 ( Fig. 2h ). These results were confirmed in immunostainings of teratoma sections, in which neural rosettes expressed NCAM but not CLDN-6 ( Fig. 2i ), whereas endodermal epithelium structures often expressed both SOX-17 and CLDN-6 ( Fig. 2j ). Taken together, these data show that CLDN-6 expression is significantly downregulated within the first few weeks of differentiation into non-endodermal tissues, but remains realatively high in the developing human endoderm (despite its absence from adult endodermal-derived tissues). These data suggest that targeting CLDN-6-positive cells might allow to purge undifferentiated cells from most hPSC-derived cell cultures. CLDN-6-based immunologic separation and elimination of hPSCs We next explored whether CLDN-6 could be used as a marker to separate undifferentiated cells from their differentiated progeny by FACS. HESCs were differentiated in a monolayer for 10 days, mixed 1:1 with their undifferentiated counterparts and then sorted by FACS ( Fig. 3a ). Only cells that were clearly high or clearly negative for CLDN-6 expression (that is, cells from both edges of the fluorescence histogram) were collected, to minimize a potential cross-contamination of these populations. To test the pluripotency of the two populations in vitro , the sorted cells were then cultured under ES cell conditions (on mouse embryonic fibroblasts, with ES medium), and pluripotent colonies could be recovered only from the CLDN-6-positive population ( Fig. 3b ). To test their pluripotency in vivo , the two populations were injected subcutaneously into immune-compromised mice. Each mouse was injected with CLDN-6-positive cells into one side of its body and CLDN-6-negative cells into the other side. Importantly, the same total number of cells was injected into both sides. In our model system, it is essential that under control conditions teratomas will be formed in 100% of the cases. It was previously reported that ~1 × 10 6 undifferentiated cells need to be injected subcutaneously to achieve this aim [4] , and this estimation holds true in our hands. We thus used this cell number for transplantation in our teratoma experiments. Mice were killed after 8 weeks, and teratoma formation was assessed. All four injected mice developed teratomas only in the side injected with CLDN-6-positive cells ( Fig. 3c ). Thus, FACS with an antibody against CLDN-6 can reduce the tumorigenicity of the cell population in our model system. 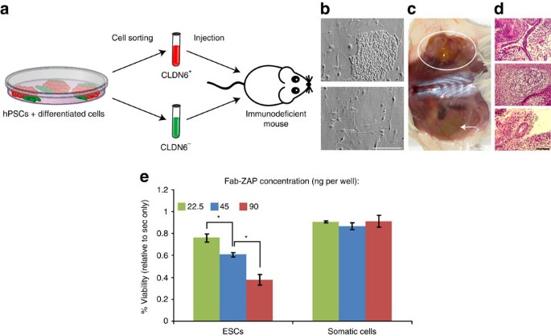Figure 3: Separation and elimination of undifferentiated cells with an anti-Claudin-6 antibody. (a) A schematic representation of the cell-sorting experiment. (b) Recovery of pluripotent colonies 1 week after cell sorting from the CLDN-6-positive cells (top) but not from the CLDN-6-negative cells (bottom). Scale bar, 100μm. (c) Teratoma formation in NOD-SCID IL2Rγ−/− mice 8 weeks after the injection of CLDN-6-positive cells (top, encircled), but not CLDN-6-negative cells (bottom, arrow). (d) Representative images of haematoxylin and eosin staining of the derived teratomas. From top to bottom: gut epithelium, cartilage and neural rosette structures are presented. Scale bar, 100 μm. (e) Relative viability of undifferentiated and differentiated cells 72 h after exposure to primary mouse IgG anti-human CLDN-6 antibody and secondary saporin toxin-conjugated anti-mouse IgG antibody. Viability of hESCs was dependent on the concentration of the cytotoxic antibody, with significant reduction between first and second concentrations (*P=0.018 by Student’st-test) and between second and third concentrations (*P=0.013 by Student’st-test). Error bars indicate s.d. of the mean.n=3. Figure 3: Separation and elimination of undifferentiated cells with an anti-Claudin-6 antibody. ( a ) A schematic representation of the cell-sorting experiment. ( b ) Recovery of pluripotent colonies 1 week after cell sorting from the CLDN-6-positive cells (top) but not from the CLDN-6-negative cells (bottom). Scale bar, 100μm. ( c ) Teratoma formation in NOD-SCID IL2Rγ−/− mice 8 weeks after the injection of CLDN-6-positive cells (top, encircled), but not CLDN-6-negative cells (bottom, arrow). ( d ) Representative images of haematoxylin and eosin staining of the derived teratomas. From top to bottom: gut epithelium, cartilage and neural rosette structures are presented. Scale bar, 100 μm. ( e ) Relative viability of undifferentiated and differentiated cells 72 h after exposure to primary mouse IgG anti-human CLDN-6 antibody and secondary saporin toxin-conjugated anti-mouse IgG antibody. Viability of hESCs was dependent on the concentration of the cytotoxic antibody, with significant reduction between first and second concentrations (* P =0.018 by Student’s t -test) and between second and third concentrations (* P =0.013 by Student’s t -test). Error bars indicate s.d. of the mean. n =3. Full size image As cell sorting may not be an optimal procedure for some types of clinical applications (for example, when single cells are not suitable for transplantation), an alternative strategy to remove hPSCs from culture may be their elimination by CLDN-6-specific cytotoxic antibodies. It has been previously suggested that Claudins may be used as targets for carcinoma therapy, and antibodies against Claudins were shown to destroy tumours that express them [24] . To address this issue, we used secondary cytotoxic antibodies that target and eliminate cells that recognize a primary antibody of interest [25] . HPSCs and fully differentiated cells (BJ fibroblasts) were exposed to mouse monoclonal IgG antibody against CLDN-6, together with a saporin toxin-conjugated anti-mouse IgG antibody (Fab-ZAP), and the viability of the cells was evaluated after 72 h. Although no change in the viability of differentiated cells was detected following their exposure to the antibodies, the same exposure induced massive cell death in the undifferentiated cells, with as much as ~70% reduction in cell viability ( Fig. 3e ). Although such a reduction is clearly not sufficient to guarantee teratoma prevention, these results demonstrate the usefulness of CLDN-6 for immunologic elimination of hPSCs, and call for the development of a toxin-conjugated primary antibody against CLDN-6. CPE selectively kills hPSCs and prevents teratoma formation We next sought to develop a chemical approach for efficiently attacking CLDN-6-expressing cells. For that aim, we investigated the usefulness of Clostridium perfringens enterotoxin (CPE), a potent toxin that specifically binds to several members of the Claudin family, leading to massive changes in membrane permeability that result in rapid cell death [26] . CPE is known to target six of the Claudin family members, including CLDN-6, and we therefore hypothesized that it can be used to eliminate undifferentiated cells from culture. Remarkably, we found that hPSCs are extremely sensitive to CPE: a short 1-h exposure of the cells to the toxin induced cell death of practically all cells in culture, whereas the same exposure did not induce any cell death in fibroblasts, which are mesenchymal cells that do not express Claudins ( Fig. 4a ). The high sensitivity of hPSCs to CPE is probably due to high expression not only of CLDN-6, but also of two other CPE-targeted Claudins (namely, CLDN-3 and CLDN-7), in these cells ( Supplementary Fig. S1a ). 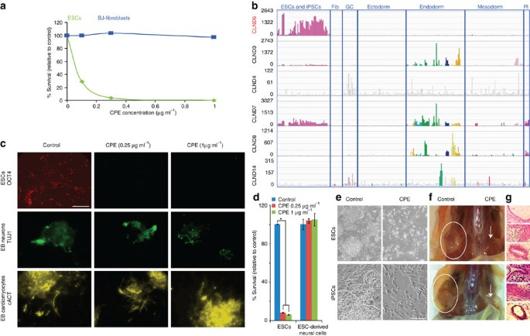Figure 4: CPE selectively kills undifferentiated cells and prevents teratoma formation. (a) Relative viability of undifferentiated hESCs and differentiated human fibroblasts 1 h after exposure to increasing concentrations of CPE, as measured by methylene blue staining. (b) Expression of the six CPE-bound Claudins in various embryonic and adult human tissues (based on Amazonia expression atlas visualization; probesets 203953_s_at, 1569421_at, 208474_a, 202790_at, 214598_at and 210689_at are presented for CLDN-3, CLDN-4, CLDN-6, CLDN-7, CLDN-8 and CLDN-14, respectively). Fib, fibroblasts; GC, germ cells; Pl, placenta. Ectoderm, mesoderm and endoderm include many cell types, as detailed inFig. 1b. (c) Fluorescence microscopy imaging of undifferentiated H9 hESCs (upper panel), differentiated neurons (central panel) and differentiated cardiomyocytes (lower panel) after 1-h exposure to CPE (at 0, 0.25 or 1 μg ml−1). Scale bar, 100 μm. (d) Relative viability of undifferentiated hESCs and of neural progenitor cells differentiated from hESCs 1 h after exposure to CPE, as measured by methylene blue staining. Error bars indicate s.d. of the mean.n=3. *P<0.01 by Student's t-test. (e) Light microscopy imaging of mixed populations of undifferentiated and differentiated cells exposed to CPE (1 h, 1 μg ml−1) or to control conditions. Scale bar, 100 μm. (f) Teratoma formation in NOD-SCID IL2Rγ−/− mice 6 weeks after the injection of mixed cell populations. Only the control cells generated teratomas (left side, encircled), whereas the injected CPE-treated cells did not (right side, arrow). (g) Representative images of haematoxylin and eosin staining of the derived teratomas. From top to bottom: gut epithelium, skeletal muscle and neural rosette structures are presented. Scale bar, 100 μm. Figure 4: CPE selectively kills undifferentiated cells and prevents teratoma formation. ( a ) Relative viability of undifferentiated hESCs and differentiated human fibroblasts 1 h after exposure to increasing concentrations of CPE, as measured by methylene blue staining. ( b ) Expression of the six CPE-bound Claudins in various embryonic and adult human tissues (based on Amazonia expression atlas visualization; probesets 203953_s_at, 1569421_at, 208474_a, 202790_at, 214598_at and 210689_at are presented for CLDN-3, CLDN-4, CLDN-6, CLDN-7, CLDN-8 and CLDN-14, respectively). Fib, fibroblasts; GC, germ cells; Pl, placenta. Ectoderm, mesoderm and endoderm include many cell types, as detailed in Fig. 1b . ( c ) Fluorescence microscopy imaging of undifferentiated H9 hESCs (upper panel), differentiated neurons (central panel) and differentiated cardiomyocytes (lower panel) after 1-h exposure to CPE (at 0, 0.25 or 1 μg ml −1 ). Scale bar, 100 μm. ( d ) Relative viability of undifferentiated hESCs and of neural progenitor cells differentiated from hESCs 1 h after exposure to CPE, as measured by methylene blue staining. Error bars indicate s.d. of the mean. n =3. * P <0.01 by Student's t-test. ( e ) Light microscopy imaging of mixed populations of undifferentiated and differentiated cells exposed to CPE (1 h, 1 μg ml −1 ) or to control conditions. Scale bar, 100 μm. ( f ) Teratoma formation in NOD-SCID IL2Rγ−/− mice 6 weeks after the injection of mixed cell populations. Only the control cells generated teratomas (left side, encircled), whereas the injected CPE-treated cells did not (right side, arrow). ( g ) Representative images of haematoxylin and eosin staining of the derived teratomas. From top to bottom: gut epithelium, skeletal muscle and neural rosette structures are presented. Scale bar, 100 μm. Full size image These intriguing results led us to examine which cell types do not express any of the Claudins bound by CPE, and may thus be resistant to this toxin. A gene expression comparison revealed that many cell types, including most mesenchymal and ectodermal cells, do not express the CPE-sensitive Claudins ( Fig. 4b ). Many of these cell types, such as neurons, cardiomyocytes and blood cells, are clinically relevant. We generated EBs from hESCs and let them spontaneously differentiate for 21 days. EBs were then dissociated and cells were replated in a monolayer. Neuronal cells were immunostained with an antibody against TUJ-1, and cardiomyocytes were immunostained with an antibody against cardiac-actin. As expected, no significant change in the viability of neurons and cardiomyocytes was observed following CPE exposure ( Fig. 4c ), in a sharp contrast to the total elimination observed in the undifferentiated cell population ( Fig. 4a ). To quantify this differential effect of CPE exposure, hESCs were differentiated to neural progenitor cells using a previously described differentiation protocol [27] , exposed to CPE and the number of viable cells was quantified; in sharp contrast to the robust cytotoxicity of CPE towards undifferentiated hPSCs, the viability of hPSC-derived neural cells was not affected by the toxin ( Fig. 4d ). Finally, to examine whether CPE can be used to prevent teratoma formation, hESCs were differentiated for a 10-day period, mixed in 1:1 ratio with their undifferentiated counterparts and the cell mixture was then exposed to CPE. Alternatively, hiPSCs were mixed in 1:1 ratio with their fibroblasts of origin and the cell mixture was then similarly exposed to CPE ( Fig. 4e ). Cells were then injected subcutaneously into NOD-SCID IL2Rγ−/− mice, so that each mouse was injected with control cells into one side of its body and with treated cells into the other side. Importantly, the same total number of cells (~1 million) was injected into both sides. We mixed undifferentiated cells with their differentiated progeny, rather than transplanting differentiated cultures per se , to ensure teratoma formation under control conditions. This approach is well accepted in the field [5] , [13] , [28] , as transplantation of differentiated cultures results in a low prevalence of teratoma formation [4] , [6] , [29] , which considerably complicates statistical analysis. Mice were killed 6 weeks later, and teratoma formation was assessed. All four injected mice developed teratomas only in the side injected with the control cells, whereas no teratomas formed in the side injected with CPE-treated cells ( Fig. 4f ). To examine what happens to the transplanted cells when no teratoma is formed, the site of injection was explanted, sectioned and stained by haematoxylin and eosin or by an antibody against human nuclei. No human cells could be detected, indicating that the cell grafts were possibly washed away from the injection site ( Supplementary Fig. S3a,b ). We next wanted to verify that CPE treatment really prevents teratoma formation, rather than just delays it. For that aim, we transplanted CPE-treated hESCs into three more mice, and teratoma formation was assessed 12 weeks after the injection. No sign for teratoma formation was observed in these long-term experiments ( Supplementary Fig. S3c ). Lastly, to examine the applicability of CPE-based elimination of undifferentiated cells in a directed differentiation model system, hESCs were differentiated to neural progenitor cells using a previously described differentiation protocol [27] , mixed in 1:1 ratio with their undifferentiated counterparts, and the cell mixture was then exposed to CPE. Cells were then injected subcutaneously into NOD-SCID IL2Rγ−/− mice, so that each mouse was injected with control cells into one side of its body and with treated cells into the other side. All four injected mice developed teratomas only in the side injected with the control cells, whereas no teratomas formed in the side injected with CPE-treated cells ( Supplementary Fig. S3d ). We therefore conclude that CPE can be used to eliminate undifferentiated cells and prevent teratoma formation, and that this strategy can be applied to remove residual undifferentiated cells from cultures of clinically relevant cell types. hPSCs are a promising source of cells for regenerative medicine because of their unique self-renewal and differentiation properties. However, the same traits that enable them to self-renew also enable them to generate tumours, and thus hinder the use of hPSC-derived cells in cell therapy. For the safe use of hPSCs in the clinic, residual undifferentiated cells must be eliminated from differentiated cultures before their transplantation. In this work, we identified the tight-junction protein CLDN-6 as a highly specific cell surface marker of hPSCs. During hPSC differentiation, CLDN-6 is rapidly downregulated, but it is still expressed in developing endodermal epithelium, in line with previous findings [20] Therefore, we expect that CLDN-6 antibody-based targeting of residual undifferentiated hPSCs could be carried out early on during differentiation towards ectodermal and mesodermal cell types, but might not be applicable to some endodermal differentiation protocols (until later stages of differentiation, when the cells should become more similar to mature adult cells that do not express CLDN-6). The use of CPE, which targets several Claudin family members, is also restricted to separating hPSCs from non-epithelial cells (thus ruling out its potential use in most endodermal differentiation protocols). Importantly, however, many clinically relevant cell types do not express these Claudins, and we experimentally validated that hPSC-derived neurons and cardiomyocytes are not targeted by CPE, so that hPSCs could be selectively eliminated from such differentiated cultures. Another advantage of CPE is that targeting several Claudins simultaneously precludes a potential selection for rare CLDN-6-negative undifferentiated cells, which might arise if one targets CLDN-6 alone. Of note, while small molecules can also selectively eliminate undifferentiated hPSCs from culture [30] , CPE-based elimination is much faster and is exerted through a well-characterized mechanism of action. In conclusion, we explored various strategies for the elimination of hPSCs from culture based on CLDN-6 expression: separation of CLDN-6-positive cells from culture by FACS; selective targeting of hPSCs by a conjugated cytotoxic antibody; and selective elimination of hPSCs by the toxin CPE. We found that CLDN-6 targeting can remove hPSCs from culture in a rapid, robust and efficient manner, thus preventing teratoma formation from undifferentiated cells. This work provides a proof of concept for the use of CLDN-6 to eliminate residual undifferentiated hPSCs from culture. It also presents a successful chemical approach to ablate these tumorigenic cells and prevent them from generating tumours. We thus expect these results to increase the safety of hPSC-based cell therapies, facilitating the use of hPSC-derived cells in regenerative medicine. Cell culture HESC lines, H9 (ref. 31 ) and CSES2-SO2/3 (ref. 32 ), BJ fibroblasts and FS fibroblasts, and hiPSC lines BJ-iPS28, BJ-iPS29 and FS-iPS1 (ref. 33 ), were cultured as previously described [33] . In-vitro differentiation in a monolayer was performed for a period of 10–14 days, by withdrawal of basic fibroblast growth factor from the growth media. Retinoic acid (Sigma-Aldrich) was added to the medium at a final concentration of 1 μM. In-vitro differentiation into EBs was performed by withdrawal of basic fibroblast growth factor from the growth media and allowing aggregation in Petri dishes as previously described [31] . In-vitro differentiation into neural progenitor cells was performed as previously described [27] . Global gene expression analysis The following cell types were subjected to gene expression microarrays: hESCs, hiPSCs, 30- and 21-day-old EBs differentiated from hiPSCs, and the fibroblasts used for the hiPSC derivation. Total RNA was extracted using PerfectPure RNA Cultured Cell Kit (5 Prime; Fisher, Waltham, MA), according to the manufacturer’s protocol. RNA was subjected to Human Gene 1.0 ST Array platform (Affymetrix); washing and scanning were performed according to the manufacturer’s protocol. Reference gene expression data from 11 human adult tissues were downloaded from the manufacturer’s website ( http://www.affymetrix.com/support/technical/sample_data/ gene_1_0_array_data.aff). Arrays were normalized using RMA algorithm in the Affymetrix Expression Console. Using a 10-fold threshold and the cellular component gene ontology (GO annotation), a list of cell surface genes differentially expressed between undifferentiated hPSCs and adult tissues was comprised. Immunocytochemistry For immunocytochemistry staining, cells were washed twice with PBS, fixed with 4% paraformaldehyde for 10 min at room temperature (RT), permeablized with 0.1% Triton X-100 and blocked in 2% bovine serum albumin in PBS for 1 h. Staining with primary antibodies was performed with the following antibodies (diluted in blocking solution): mouse anti-human OCT-3/4 (IgG, 1:200; Santz Cruz Biotechnology), rabbit anti-human OCT-3/4 (IgG, 1:200, Santz Cruz Biotechnology), mouse anti-human CLDN-6 (IgG, 1:40, R&D Systems), mouse anti-human TUJ-1 (IgG, 1:1,000; Sigma-Aldrich), mouse anti-human cardiac-actin (IgG, 1:200; Maine Biotechnology Services), goat anti-human SOX-17 (IgG 1:400, R&D Systems) and mouse anti-human nuclei (IgG, 1:100, Chemicon). Cells were incubated for 1 h at RT with primary antibody, washed, and incubated with conjugated secondary antibodies at RT (Jackson Immunoresearch laboratories) for another 1 h. Staining with Hoechst 33342 (Invitrogen) was used to detect the nuclei. FACS analysis and cell sorting Colabeling of CLDN-6 with known pluripotency markers was performed on ice with mouse anti-human CLDN-6 antibody (IgG, 1:40, R&D Systems), together with either rat anti-human SSEA-3 antibody (IgM, 1:100, Chemicon) or mouse anti-human TRA-1-60-PE antibody (IgG, 1:40, BD Biosciences). Cells were washed and incubated when appropriate with secondary antibodies: FITC-conjugated goat anti-mouse IgG (1:200, Jackson Immunoresearch laboratories), FITC-conjugated donkey anti-mouse (1:200, Jackson Immunoresearch laboratories) and Cy5-conjugated donkey anti-rat (1:200, Jackson Immunoresearch laboratories). Analysis was performed using FACSAria Cell-Sorting System (Becton Dickinson). For analysis of pluripotency after knockdown, cells were incubated on ice with TRA-1-60-PE antibody (1:40, BD Biosciences), washed and analysed using LSR_II FACS (BD Biosciences) with FCS Express software ( De Novo Software). For quantification of apoptosis after knockdown, Annexin V-FITC Apoptosis Detection Kit (eBioscience, San Diego, CA) was used, according to the manufacturer’s instructions. Analysis was performed using FACSAria Cell-Sorting System (Becton Dickinson). The cell cycle analysis was performed using propidium iodide staining. Cells were trypsinized and incubated in methanol at −20 °C for 2 h. RNA digestion was performed with 200 μg ml −1 RNase A (Sigma-Aldrich) for half an hour at RT. Cells were stained with 50 μg ml −1 propidium iodide for 10 min at 25 °C, and were taken for FACS analysis. Analysis was performed using FACSAria Cell-Sorting System (Becton Dickinson). For cell sorting, cells were incubated on ice with mouse anti-human CLDN-6 antibody (IgG, 1:40, R&D Systems), washed and incubated with FITC-conjugated goat anti-mouse IgG antibody (1:200, Jackson Immunoresearch laboratories), and cell sorting was performed using FACSAria Cell-Sorting System (Becton Dickinson; 100-μm nozzle with low pressure). RNA isolation and quantitative real-time PCR Total RNA was extracted using PerfectPure RNA Cultured Cell Kit (5 Prime). One microgram of total RNA was used for reverse transcription reaction using ImProm-II reverse transcriptase (Promega). Quantitative real-time PCR was performed with 1 μg of RNA reverse transcribed to complementary DNA and TaqMan Universal Master Mix or Power SYBR Green PCR Master Mix (Applied Biosystems), and analysed with the 7300 real-time PCR system (Applied Biosystems). Primer sequences for CLDN-6 are: 5′-GGAATGCAGATCCTGGGAGT-3′ (forward) and 5′-ATGAAAGCGGTCACCTTCC-3′ (reverse); Taqman probes for OCT-4, REX-1 and GAPDH are: Hs 03005111_g1, Hs 00233521_m1 and Hs99999905_m1 (respectively). Knockdown of CLDN-6 To knockdown CLDN-6 in hESCs, ON-TARGETplus SMART pool short interfering RNA against human CLDN-6 (Dharmacon RNAi Technologies) was transfected into the cells. Transfection was performed as previously described [34] , using the transfection reagent Lipofectamine 2000 (Invitrogen). Cells were collected and RNA was extracted 72 h after transfection. Cell viability assays Relative cell numbers were determined by fixating the cells with 0.5% glutardialdehyde (Sigma-Aldrich) and staining with methylene blue (Sigma-Aldrich) dissolved in 0.1 M boric acid (pH 8.5). Colour extraction was performed using 0.1 M hydrochloric acid, and the staining (which is proportional to cell number) was quantitated by measuring absorbance at 650 nM. Fluorescence microscopy and image analysis Images were taken using an Olympus IX81 microscope with MT20/20 illumination system and aC10600-10B Hamamatsu camera. For high-content image analysis, multiple images were taken automatically using the ScanR acquisition system. Image analysis and quantification was then performed using the ScanR analysis software. Teratoma section images were taken on an Olympus IX70 mounted with a DP71 camera. Confocal imaging was performed using an MRC-1024 Bio-Rad confocal scan head coupled to a Zeiss Axiovert 135M inverted microscope. CPE assay CPE was purchased from Abcam, and treated according to the manufacturer’s instructions. Cells were exposed to CPE, diluted in their culture medium, for 1 h at RT before cell viability or teratoma formation assays. Teratoma formation For expression microarray experiments, undifferentiated hiPSCs were collected with trypsin–EDTA (Biological Industries) and counted using Countess automated cell counter (Invitrogen). Approximately 3 × 10 6 cells were resuspended in ES medium to a total volume of 200 μl. Cells were then injected into the kidney capsule of NOD-SCID mice. Four weeks after injection mice were killed, the formation of tumours was examined and the resulting teratomas were photographed, dissected and cryopreserved in OCT compound (Sakura Finetek). Histological slides were fixed in 100% methanol for 10 min at −20 C, and stained with haematoxylin and eosin. For cell-sorting experiments, hESCs were differentiated for 10 days, as described above, and were then collected, mixed at a 1:1 ratio with their undifferentiated parental, stained with anti-human CLDN-6 antibody and sorted as described above. Cells were thus sorted to CLDN-6-positive and CLDN-6-negative populations. 0.75 × 10 5 viable cells from each population were resuspended in 1:1 ES medium:matrigel to a total volume of 200 μl. Cells were then injected subcutaneously to the back of NOD-SCID IL2Rγ−/− mice. Each mouse was injected with CLDN-6-positive cells into one side of its body and CLDN-6-negative cells into the other side. Eight weeks after injection mice were killed, tumour formation was examined and teratomas were treated as described above. For CPE experiments, hESCs were differentiated for 10 days, as described above, or using a neural differentiation protocol [27] , and were then collected and plated at a 1:1 ratio with their undifferentiated parental cells in six-well tissue culture plates (Cellstar). Alternatively, hiPSCs were collected and plated at a 1:1 ratio with their fibroblasts of origin in six-well tissue culture plates. Twenty-four hours later, cells were exposed either to CPE (1 μg ml −1 ) or to 0.25% DMSO for 1 h, and were then collected and counted. A total of 1 × 10 6 viable cells from each condition were resuspended in 1:1 ES medium:matrigel to a total volume of 200 μl. Cells were then injected subcutaneously to the back of NOD-SCID IL2Rγ−/− mice. Each mouse was injected with CPE-treated cells into one side of its body and control-treated cells into the other side. Six or twelve weeks after injection mice were killed, tumour formation was examined and teratomas were treated as described above. All experimental procedures were approved by the ethics committee of the Hebrew University. Statistics P -values were determined by one-tailed Student’s t -test. N =3 in RT–PCR and cell viability experiments. Accession codes: HESC and hiPSC microarray data have been deposited in NCBI Gene Expression Omnibus (GEO) under the accession codes GSE21244 and GSE38088 . How to cite this article: Ben-David, U. et al. Immunologic and chemical targeting of the tight-junction protein Claudin-6 eliminates tumorigenic human pluripotent stem cells. Nat. Commun. 4:1992 doi: 10.1038/ncomms2992 (2013).